Nanoscale light–matter interactions in atomic cladding waveguides Alkali vapours, such as rubidium, are being used extensively in several important fields of research such as slow and stored light nonlinear optics quantum computation, atomic clocks and magnetometers. Recently, there is a growing effort towards miniaturizing traditional centimetre-size vapour cells. Owing to the significant reduction in device dimensions, light–matter interactions are greatly enhanced, enabling new functionalities due to the low power threshold needed for nonlinear interactions. Here, taking advantage of the mature platform of silicon photonics, we construct an efficient and flexible platform for tailored light–vapour interactions on a chip. Specifically, we demonstrate light–matter interactions in an atomic cladding waveguide, consisting of a silicon nitride nano-waveguide core with a rubidium vapour cladding. We observe the efficient interaction of the electromagnetic guided mode with the rubidium cladding and show that due to the high confinement of the optical mode, the rubidium absorption saturates at powers in the nanowatt regime. Light–matter interactions with alkali vapours have been the subject of a flourishing research field for several decades. In addition to providing basic information on the properties of these atoms, such interactions hold grand promises for a variety of applications spanning from the control of speed of light by the slow and fast light effects [1] , [2] , few-photon switching [3] and quantum computation [4] , [5] to frequency stabilization [6] , and magnetometry [7] . Currently, alkali vapours such as rubidium (Rb) and caesium (Cs) are already serving as key components in modern navigation and communication [8] , [9] . Following the general trend for miniaturization and high-level integration, there is an ongoing effort towards tightly confining light and vapour in order to obtain efficient, miniature and low-power light–vapour interactions. Recent works demonstrated significant reduction in the interaction volume by the use of micro and nano vapour cells [10] , [11] , [12] . In parallel, several works demonstrated the interaction of thermal alkali vapours with light in guided mode configuration. This includes the use of hollow core photonic crystal fibres [13] , [14] , [15] , [16] (HC-PCFs), hollow core anti-reflecting optical waveguides [17] , [18] , [19] (HC-ARROWs), tapered nanofibres [20] , [21] , [22] (TNFs) and nano waveguides [23] . In an HC-PCF, alkali vapour is pumped into the core of the fibre and interacts with the electromagnetic field that is guided along the core of the HC-PCF. This platform served for the demonstration of a variety of effects including vapour spectroscopy [13] , [15] , electromagnetic-induced transparency [14] and enhanced two-photon absorption [16] . Alternatively, the TNF approach, consisting of solid core fibre surrounded by Rb vapour cladding, was already shown to be useful for nanowatt saturation of the atomic transition [20] , two photon absorption [21] and efficient all-optical switching [22] . A further step towards miniaturization and integration was accomplished by constructing hollow core waveguides on a chip, via the use of the HC-ARROW [18] , [19] approach. This work has the benefit of being both compact and chip-integrable, and enables strong light–matter interaction on chip. The ability to achieve electromagnetic-induced transparency and consequently slow light in this platform has been further demonstrated [19] . In spite of the fact that the HC-ARROW concept provides an important step towards miniaturization and integration, reducing the dimensions of the guided mode towards the submicron regime remains an immense challenge. In this work, we tackle this challenge by establishing an on-chip platform for strong light-matter interactions in a chip-scale environment by using a solid core waveguide surrounded by Rb vapour cladding. This configuration can be considered as the on-chip equivalent of the TNF approach, where the evanescent tail of the electromagnetic mode interacts with the alkali vapour. A natural choice of platform for the realization of the solid core waveguide in the submicron regime is that of the silicon photonics, which enables strong light confinement and dense integration of devices on a chip. Indeed, the emerging field of silicon photonics is becoming a key technology in the construction and the demonstration of various nanoscale devices for myriad applications such as communication, signal processing and sensing, to name a few [24] , [25] . Unfortunately, silicon core waveguides cannot be used for the interaction of light with Rb or Cs atoms because of their lack of transparency in the relevant spectral window between 770–900 nm. Yet, one can use silicon nitride (SiN) as the waveguide core material. In addition to being used routinely in the complementary metal oxide-semiconductor industry, SiN offers several prominent advantages; it is transparent both in the visible and the infrared spectrum, it possesses moderately high refractive index ( n ~2), thus allowing tight confinement of the optical mode. Additionally, being a dielectric material with large energy bandgap SiN does not suffer from free carrier’s absorption at wavelengths of >300 nm. Another advantage of SiN is its low thermo-optic coefficient (~10 −5 K −1 ), making it less sensitive to environmental variations. Following these properties, submicron SiN waveguides were recently demonstrated for sensing, filtering and nonlinear optics applications [26] , [27] , [28] , [29] . Here, we demonstrate an atomic cladding waveguide (ACWG) consisting of a SiN core nano-waveguide integrated with an alkali vapour cladding, and reveal evanescent light–matter interactions on a chip, with nanoscale dimensions and low light level interactions in both the linear and the nonlinear regime. Using this approach, one can integrate atomic vapour on top of an existing complementary metal oxide-semiconductor-compatible photonic circuit, and selectively enable the interaction of the light and atoms in arbitrary regions of the chip. For example, one can think of obtaining strong light mater interactions of Rb atoms with nanophotonic resonators, for example, micro ring/disk resonators, photonic crystal resonators as well as with on-chip nanofocusing devices [30] , [31] and nanoantennas [32] . Such a platform may also be used for achieving strong-coupling cavity quantum electrodynamics in a chip-scale environment [33] . Using this concept of ACWG, we also observed nonlinear phenomena in ultra-low levels of light. This is because of the tight confinement of light in our ACWG, having a mode area of 0.3λ 2 . Parallel to our experimental demonstration, we suggest a framework to analytically predict the absorption spectra of such ACWGs. Our model includes the specific broadening mechanism unique to our system, that is, the increased Doppler broadening and evanescent transit-time broadening. The model prediction is compared with our experimental results and found to be in good agreement. Construction of an atomic cladding waveguide Our ACWG is illustrated in Fig.1a , where a photonic chip consisting of few SiN waveguides with a silicon oxide cladding is sketched. Above a chosen region on the chip, the upper oxide cladding is etched out and a cylinder is epoxy-bonded to the chip. This opening will be used as the interaction region between the optical mode guided by the SiN waveguide and the Rb atoms. Next, the cell is connected to a vacuum system, baked out and a droplet of natural abundance Rb is inserted. In all other regions expect this interaction region, the waveguides are buried under the oxide layer. The fabrication method of such an integrated ACWG is described in the Methods. 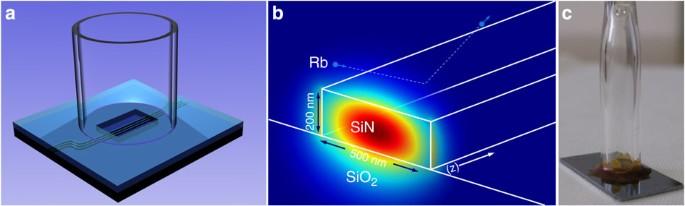Figure 1: Atomic cladding waveguide illustration and photograph. (a) Illustration of the ACWG. (b) Cross section of the SiN waveguide in the interaction area with the simulated fundamental TE mode superimposed. A Rb atom is illustrated as reflecting the surface, leaving the surface at a quenched state. (c) Photograph of the device showing the bonding of the vapour cell to the chip. Figure 1: Atomic cladding waveguide illustration and photograph. ( a ) Illustration of the ACWG. ( b ) Cross section of the SiN waveguide in the interaction area with the simulated fundamental TE mode superimposed. A Rb atom is illustrated as reflecting the surface, leaving the surface at a quenched state. ( c ) Photograph of the device showing the bonding of the vapour cell to the chip. Full size image The waveguide structure was designed to support a transverse electric (TE)-like mode, in-plane polarization with width and height of 500 and 200 nm, respectively. The waveguide dimensions were chosen as a compromise between the desire for strong light–matter interactions and dense integration, requiring high confinement of the optical mode in the waveguide core and the need for significant interaction of light with the surrounding atoms, requiring a substantial portion of the optical mode to reside in the cladding. In addition to affecting the strength of interaction, the specific geometry of the waveguide is also expected to determine the absorbance profile due to the Doppler broadening and transit-time broadening, which are affected by the propagation constant of the optical mode and the evanescent decay lengths, respectively. In Fig. 1b , we present an illustration of such a waveguide, with the simulated mode profile calculated by the finite element method (Comsol multiphysics) superimposed on it. The confinement factor of the mode, that is, the fraction of the electric field that interacts with the Rb, is found to be 10.9%, calculated by integrating the fraction of intensity in the interaction region divided by the unit input power. A Rb atom is illustrated as ballistically striking and reflecting from the surface (dark blue dashed lines). The nature of this process in the context of the absorption spectrum will be evident in the next paragraph. In Fig. 1c , a photograph of the integrated device is shown. Calculation of the effective susceptibility of an ACWG In order to calculate the effective index of refraction of the atomic cladding layer and to shed light on the dynamics of the transmission spectrum in our system, we adapt the method developed in the context of attenuated total internal reflection (ATIR). The reflection of light from an interface between a dielectric and a vapour has been investigated thoroughly, both theoretically and experimentally, and particularly in the case of total internal reflection [34] , [35] , [36] , [37] . Owing to the non-local nature of response of the atoms to the applied field, resulting from the transient response of group of atoms emanating from the surface [34] , there is a need to find an effective susceptibility that takes into account the dynamic nature of light–matter interactions as a consequence of the collision of the atoms with the wall. While calculating the effective susceptibility, one must consider the finite time of interaction. Owing to the evanescent decay of field in the vapour, the time of interaction between the atoms and the electromagnetic wave is finite, and is typically lower than the lifetime of the excited level. This effect results in broadening of the spectrum, known as the transit-time broadening. Additionally, one must consider the effect of the pseudomomentum carried by the mode along the propagation direction. This momentum results in an increase in the Doppler broadening of the absorption spectrum. In order to find the effective susceptibility, one solves the optical Bloch equations, with a boundary condition of total dephasing (quenching) when an atom hits the dielectric. The solution is separated for the steady-state solution, for the atoms moving toward the wall (transverse velocity v t <0) and a transient solution for the atoms moving from the wall (transverse velocity v t >0). Using these two solutions and the concept of the fictitious polarization, it can be shown [34] , [36] , [37] that first order susceptibility is given by the following expression: where N is the density of atoms, e the electric charge of an electron, ε 0 the vacuum permittivity, m e is the electron mass, C i is the occupation ratio, is the transition frequency from a level with total angular momentum F to an excited state with momentum F′, v z and v t are the atomic velocities in the propagation direction z and the transverse direction, respectively, W is the normalized velocity distribution, k z and k t represent the momentum of the evanescent field along the propagation direction and the transverse direction respectively. 2 γ is the natural full-width half maximum line-width and Δ ν , the frequency detuning from the transition frequency. The oscillator strengths f FF′ are defined using the different quantum numbers of the different transitions, as described in Supplementary Note 1 . Equation 1 is valid in the case of low vapour density, as in our experiments. In the case of higher densities, the formalism should be adapted in the same manner that has been done in the context of single reflection [37] . Thus, in order to calculate the effective refractive index, besides the density of atoms (equivalent to temperature), we need to find the momentum in the direction of propagation and the momentum in the direction perpendicular to the propagation, in order to obtain the exact line shape. The first will specify the amount of Doppler broadening and the latter will specify the amount of transit-time broadening. In waveguide terminology, these momenta are the effective wave number, β and the inverse evanescent decay length, η , respectively. The higher confined the mode, higher will be the β and smaller will be the η , resulting in an increase in both Doppler and transit time broadened line shape. As a result of the broadening, the contrast of the absorption line shape is expected to decrease. Further reduction in the contrast is also expected because of the reduced interaction of the electromagnetic field with the atomic vapour, resulting from the higher confinement of the mode in the solid core waveguide rather than in the atomic cladding. In order to evaluate the validity of the proposed model, we first compare it to published results of atomic cladding tapered fibres reported independently in refs 20 and 21 . In both cases, the model predicts the absorption spectrum adequately. This validity comparison is presented fully in Supplementary Note 1 . It should be noted that one can exploit the framework to more elaborate light–matter interactions, as the ATIR susceptibility has been developed in the case of pump–probe experiments [38] , as well as selection reflection in the case of dark resonances [39] . Atomic cladding waveguide spectroscopy Next, we investigated light propagation in our ACWG. For reference, we first measured the transmission spectrum obtained by illuminating the vapour cell directly, that is above the ACWG ( Fig. 2a ). In this figure, one can clearly see the distinct Doppler broadened absorption dips corresponding to both 85 Rb and 87 Rb absorption lines. For reference, we also show the eight oscillator strengths of the atomic transitions of 85 Rb (red vertical lines) and 87 Rb (blue vertical lines) in arbitrary units, where the oscillator strength is proportional to the height of the vertical line. Next, we coupled light directly to the ACWG and observed the obtained spectrum. The normalized transmission spectra of light propagating along the ACWG is shown in Fig. 2b . The results were obtained at a cell temperature of about 135 °C, corresponding to a density of 3.9 × 10 19 m −3 atoms. The signal has been attenuated in order to avoid saturation of the transitions. As can be clearly seen, in comparison with the bulk transmission, the absorption lines are broader. As mentioned earlier, this result is associated with an additional Doppler broadening due to the increased momentum in propagation direction, and also with an increase in the transit-time broadening resulting from the limited interaction time. This broadening manifests, for instance, in the total overlap of the 87 Rb F=2→F′=1 and the 87 Rb F=2→F′=2 transitions with the 85 Rb F=2→F′=2/3 transition. It should be noted that the data presented here was obtained on a course of few days. No evidence of degradation of the operation of the device has been witnessed. 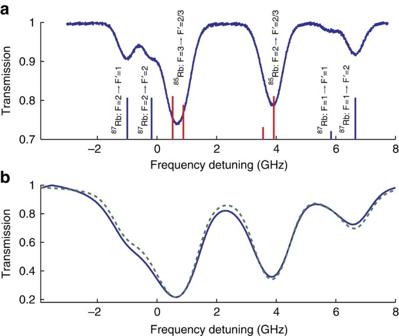Figure 2: Atomic cladding waveguide spectroscopy. (a) Natural Rb Doppler broadened spectrum, as measured through the cell attached to the silicon chip. (b) Normalized measured spectrum (blue solid line) and calculated spectrum (green dashed line). Calculations were performed based on the actual dimensions of the ACWG and the density of the vapour. Figure 2: Atomic cladding waveguide spectroscopy. ( a ) Natural Rb Doppler broadened spectrum, as measured through the cell attached to the silicon chip. ( b ) Normalized measured spectrum (blue solid line) and calculated spectrum (green dashed line). Calculations were performed based on the actual dimensions of the ACWG and the density of the vapour. Full size image In order to compare the presented model to our experimental results, we plot the simulated transmission spectrum after propagating through our ACWG ( Fig. 2b ). The spectrum is calculated based on Equation 1 using the procedure described in Supplementary Note 1 . Temperature of 135 °C, confinement factor of 0.11, interaction length of 1.5 mm, atom density of 3.9 × 10 19 m −3 , effective index of 1.56 and evanescent wave number of 9.47 × 10 6 m −1 were used to calculate this transmission spectrum. As can be seen, this model predicts both the widths and the contrast of the different absorption lines. The model predicts a broadened line resulting from a Doppler broadening of 900 MHz and transit-time broadening of 60 MHz, and an overall width of 1.1 GHz. These values were calculated by assuming no transverse velocity component (for Doppler broadening), no longitudinal velocity component (for transit-time broadening) and both velocity components (for the total width). We expect this simple model to underestimate the transit-time broadening, because it neglects the two-dimensional rectangular geometry of the problem. Transit-time broadening results reported in the literature for tapered fibre systems with optical modes having evanescent tail length comparable to our ACWG are in the range of 100–120 MHz ( [20] , [21] ). A moderate estimate of the transit-time broadening in our system in line with these measurements would be in the range of 150–200 MHz. Generally, in order to differentiate between the transit time and the Doppler broadening mechanisms, one should implement Doppler-free techniques such as saturation spectroscopy or two photon absorption. Below, we present a resonant two-photon absorption spectra, indicating a transit time broadened line smaller than ~300 MHz. The accuracy in measuring the transit-time broadening is currently limited by our samples. Future devices with lower reflection from the sample facets will provide better signal to noise ratio and are expected to further assist in determining the exact broadening values. Nonlinear interactions in the ACWG system Next, we investigated nonlinear interactions in our ACWG system. Specifically, we measured the variations in the absorption spectrum as a function of the incident light intensity. To do so, we measured the transmission spectrum with different neutral density (ND) filters set at the output of the laser, whereas the ACWG remains under constant coupling conditions and constant temperature. In Fig. 3a , we plotted the obtained transmission spectrum, whereas in Fig. 3b we plotted the contrast of the F=2→F′=2/3 transition as a function of the ND filter attenuation ratio. The actual input powers varied between 2.5 mW to 50 nW, whereas the output powers varied between 2.5 μW to 50 pW. The optical power within the waveguide was estimated by measuring the output power and taking into consideration, the coupling loss in our system. Our current version of the ACWG system is not optimized for maximum coupling efficiency. The overall coupling loss, is currently about 30 dB, including coupling loss from the fibre to the waveguide (two facets) and from the oxide-clad waveguide to the ACWG (two facets). Additionally, the epoxy glue induces some loss. These loss factors will be reduced in the future devices, for example, by increasing the thickness of the oxide-clad layer and by optimizing the dimensions of the ACWG with respect to that of the oxide-clad waveguide. By assuming a symmetric coupling scenario, we estimated the power level within the waveguide to be about 15 dB higher than the power measured at the output. We estimated the deviation from this power level to be in the range of a few dB, deduced from measuring the variations in output signal in a few different waveguides located on the same chip. 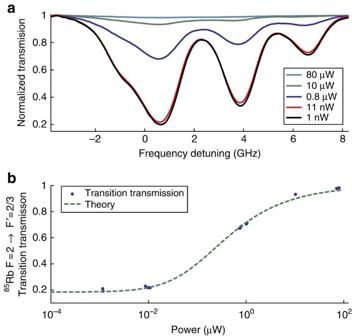Figure 3: Nonlinear interaction in an atomic cladding waveguide. (a) Normalized transmission of the ACWG with different incident power levels in the waveguide, attenuated using ND filters (b) Minimal transmission of the F=2→F′=2/385Rb transition as a function of the optical power within the ACWG. Figure 3: Nonlinear interaction in an atomic cladding waveguide. ( a ) Normalized transmission of the ACWG with different incident power levels in the waveguide, attenuated using ND filters ( b ) Minimal transmission of the F=2→F′=2/3 85 Rb transition as a function of the optical power within the ACWG. Full size image As can be clearly seen in both Figs 3a and 3b , the contrast increases with the decrease in the optical power level within the ACWG, as anticipated in a saturated transition scenario. In order to estimate the power where this saturation occurs, we fitted the data in Fig. 3b to an exponential function of the following form: T ( P )=exp(− α 0 (1+ P / P sat ) −1/2 ), where α 0 is the optical density corresponding to the unsaturated level measured, P is the optical power level within the ACWG at resonance (obtained by a linear fit around the resonance) and P sat is the saturation optical power. The square root factor is used as we expect the system to be dominant by inhomogeneous broadening. We found, using these values in Equation 2, that the estimated onset of saturation is about 40 nW. This low power level is consistent with the theoretical and experimental estimations given in refs 20 , 21 , and is the result of the high confinement of the optical mode compensating both Doppler and transit-time broadening, which increase the saturation threshold. Temperature dependence of absorption Next, we investigated the effect of temperature on the transmission of light, while the optical transitions are not saturated. 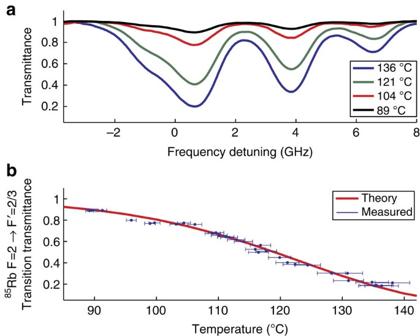Figure 4: Temperature-dependent spectroscopy. Temperature dependence of the absorption. (a) Normalized transmission of the ACWG at different temperatures. (b) Transmission of the F=2→F′=2/385Rb transition as a function of temperature, and the expected theoretical contrast using Equation 1. The error bars were calculated by measuring the thermistors resistance fluctuation at every measured point and projecting this fluctuation on the calibration curve of the thermistor. Figure 4a shows the transmission spectrum at several different temperatures. As can be noticed, the contrast increases with the increase in temperature. This is expected because higher temperatures correspond to higher densities of atoms, that is, stronger absorption. In Fig. 4b , the calculated (using Equation 1) and the measured contrast of the F=2→F′=2/3 85 Rb transition as a function of temperature are shown. Both curves are in good agreement. It is worth noticing that the absorption is achieved by the interaction of a relatively small number of atoms and photons. Calculation of the amount of atoms that interact with the optical mode, at any instant of time, can be performed by the multiplication of the evanescent volume and the density of atoms. Such calculations indicate that only a few hundred of atoms interact with the photons at the 100 °C temperature range, and a few thousand atoms at the 130 °C temperature range. Figure 4: Temperature-dependent spectroscopy. Temperature dependence of the absorption. ( a ) Normalized transmission of the ACWG at different temperatures. ( b ) Transmission of the F=2→F′=2/3 85 Rb transition as a function of temperature, and the expected theoretical contrast using Equation 1. The error bars were calculated by measuring the thermistors resistance fluctuation at every measured point and projecting this fluctuation on the calibration curve of the thermistor. Full size image Doppler-free two-photon absorption measurements Finally, in order to differentiate between Doppler broadening and other broadening mechanisms such as transit-time broadening, one should implement a Doppler-free technique. It is common practice to do so by using saturation spectroscopy, where a strong pump beam counter propagates a weaker probe beam, and by doing so, isolates the zero Doppler group velocity. As our device has not been optimized in terms of coupling efficiency, such counter-propagating experiments are quite demanding, because the back reflection masks the probe signal. When dealing with a pump–probe experiment with both the pump and the probe tuned to the same wavelength (as used in the saturation spectroscopy method), this back reflection interferes with the probe and might mask out the signal. This difficulty may be eliminated by using the Doppler-free counter propagating two-photon resonant transition [40] , in which the interference term is filtered out by the detector and the remaining pump reflectance can be filtered using a band pass filter. Such an arrangement is described in Fig. 5a , showing schematics of a counter-propagating pump–probe scheme for a resonant two-photon excitation. In this scheme, we inverted the role of the pump and the probe, as is used in the double resonance optical pumping (DROP) method [41] . Here, we monitor the variations in transmission of light at the wavelength of 780 nm, which is aligned with the 85 Rb F=3→F′=3 transition, as a result of applying a pump signal at a wavelength of ~776 nm. This is achieved by demodulating the amplitude-modulated 780-nm source. Our ACWG configuration is characterized by a short transit of the atom in the evanescent field, in the order of 1 ns. This transit time is shorter than the lifetimes of the relevant transitions, and thus the atom is not expected to relax to other levels as in the case of DROP experiments [41] . Owing to the above, the F=3→F′=3 population difference is expected to decrease, resulting in an enhanced absorption. 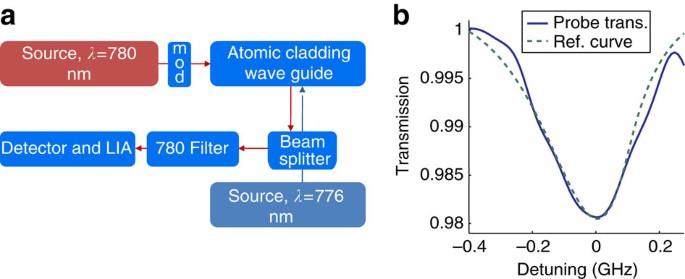Figure 5: Two-photon absorption in an atomic cladding waveguide. (a) Optical setup for measuring two-photon absorption in an atomic cladding waveguide. Mod, amplitude modulator; LIA, lock in amplifier (b) Measured transmission spectrum of the 780-nm source while being scanned by the 776-nm source (blue line), and the corresponding theoretical reference curve (green dashed line). Figure 5: Two-photon absorption in an atomic cladding waveguide. ( a ) Optical setup for measuring two-photon absorption in an atomic cladding waveguide. Mod, amplitude modulator; LIA, lock in amplifier ( b ) Measured transmission spectrum of the 780-nm source while being scanned by the 776-nm source (blue line), and the corresponding theoretical reference curve (green dashed line). Full size image Indeed, we observed this expectation experimentally. Figure 5b shows the measured transmission of the 780-nm signal as a function of the detuning of the 776-nm signal. One can clearly see a drop in the transmission, with a full-width half-maximum of 300 MHz, much below the linewidth of ~1.1 GHz measured in the single-beam spectroscopy experiment. For reference, we plotted the theoretical absorption profile, calculated by the convolution between the two photon absorption profile under a transit time broadened scenario (given by the function exp(−|Δ ν |/(Δlog4)) as in ref. 42 , with a width approximated as 150 MHz) and the time response of our measurement system. The latter is due to a technical limitation of our system being able to measure with resolution of ~100 MHz. In the future, we will demonstrate an integrated on-chip saturation spectroscopy as well as resonant two-photon absorption, using a ACWG chip specifically designed for this purpose. Such a setup will allow us to further investigate the various broadening mechanisms more accurately and thoroughly. In this paper, we have developed and presented a chip-scale platform providing efficient evanescent light–matter interactions in an atomic cladding waveguide (ACWG). Based on this platform, we demonstrated the interaction of an on-chip nanoscale-guided optical mode with Rb atoms in both the linear and the nonlinear regime. Specifically, we show the transmission spectrum of light passing through our device at various optical power levels and various temperatures. From the obtained results, we have estimated the saturation to be in the nanowatt regime. This relatively low value is the result of the high mode confinement compensating both Doppler and transit-time broadening which increase the saturation threshold. Additionally, based on the ATIR formalism, which also takes into account Doppler and transit-time broadening, we have developed a model that allows calculation of the transmission spectrum in our ACWG structures. Finally, we have also demonstrated a resonant two-photon absorption spectra, from which, the Doppler and the transit-time broadening could be separated. The results show that the Doppler broadening seems to be dominant over the transit-time broadening. The platform of ACWG offers several prominent advantages. Dimension-wise, an ACWG, has a mode area that is about two orders of magnitude smaller than previously demonstrated by on-chip approaches [17] . In addition, due to the ability to integrate large varieties of existing photonic circuits with the ACWG, this approach can further enhance light–matter interaction via the use of resonators such as micro-ring resonators and photonic crystal resonators, and structures such as slot waveguides make this platform attractive for nonlinear optics. Owing to the small mode volume achievable with our platform, one can expect an enhanced cooperativity compared with free space configurations. The ACWG SiN platform further enables to couple broadband optical signals, making it applicable (simultaneously) to various alkali vapours such as Cs and Rb and various optical transitions like the D1 and D2 lines, or higher excited Rydberg states [43] . Similar to other systems that exhibit strong light–matter interactions with atomic vapour, the ACWG is limited in the obtainable absorption line widths due to finite time of interaction and increased Doppler broadening. The latter can be reduced using various Doppler-free excitation schemes, resulting in a transit time broadened line, which can be viewed as an effective homogeneous broadening that limits the systems coherence. This, for instance, will determine the modulation frequency in switching applications [22] , [44] and the stability of an optical frequency standard, and may be decreased using a buffer gas [22] . Nevertheless, due to the unprecedented ability to control the electromagnetic field distribution in nanoscaled structures, this approach makes possible, the conduct of controlled and efficient light–matter interactions at the nanoscale, which are very challenging to be achieved in other configurations. These exciting opportunities manifest in both well-established and new applications such as few-photon switching, quantum gates and logic, slow and fast light and optical frequency standards, all in a chip-scale footprint. Finally, although this paper deals with hot atoms, the demonstrated platform may also be implemented in applications involving cold atoms, for example, cavity QED, and exploiting the chip for optical traps of atoms, taking advantages of the strong gradient of the evanescent electromagnetic field [45] , [46] , [47] . Fabrication To construct the device, we used a silicon substrate with thermally grown 2.5-μm thick silicon oxide and low-pressure chemical vapour deposited (LPCVD) 200-nm thick silicon nitride (SiN) device layer atop (Rogue Valley Microdevices). After cleaning in Piranha solution (a mixture of sulphuric acid (H 2 SO 4 ) and hydrogen peroxide (H 2 O 2 ), in 3:1 ratio), the SiN waveguides were defined using standard electron-beam lithography (Raith e-line 150) with 20 kV acceleration voltage and ZEP-520 A as a positive tone electron-beam resist (resist thickness was set to 300 nm). The lithography was followed by inductively coupled reactive ion etching ICP RIE (Oxford Plasmalab 100, Oxford Instruments) with a CHF 3 /O 2 gas mixture to transfer the pattern into the SiN device layer. After etching, the optical structure was covered with 1.5-μm thick silicon oxide layer using plasma-enhanced chemical vapour deposition (PECVD). In order to construct an atomic cell, we carried out an additional lithographic step to define a chamber area where PECVD oxide layer was later on etched down with buffered hydrofluoric acid (BHF) to expose the waveguides structure for interaction with rubidium vapour. Next, the chip was diced to its final dimensions of 1 × 2 cm. Finally, a Pyrex cylinder was bonded to the chip using thermally cured epoxy. The cell is connected to a turbo vacuum system, and baked out simultaneously. The device was baked out for 24 h, after which, a vacuum level of ~10 −8 Torr was reached. At this stage, natural Rb was launched into the cell, and then, the cell was disconnected and sealed. We have tested our device for more than half a year and it still seems to be working properly. Setup A 795 nm DFB (Toptica DL100, Toptica) source was fibre-coupled to a single-mode polarization-maintaining lensed fibre. The polarization direction was set to be aligned with the in-plane (TE) polarization mode of the ACWG. The light was coupled from the lensed fibre into the waveguide in a butt-coupling configuration. Symmetrically, light was coupled out of the waveguide into a second lens fibre using a butt-coupling configuration and the intensity was measured using a photodetector (Newport 2151, Newport or Thorlabs DET100A, Thorlabs). The intensity of the launched light was controlled by inserting ND filters at the output of the laser. In addition, a beam splitter was introduced in the output of the laser in order to measure a reference cell or the bulk of the cell attached to the waveguide simultaneously to the waveguide measurement. In order to achieve sufficient density of atoms, the device was heated using resistor heaters and the temperature was monitored using a thermistor. The thermistor is located a few millimetres away from the top of the cell. In order to reduce the accumulation of Rb on the surface of the waveguides, we maintained a temperature gradient between the top of the cylinder and the surface of the chip. This way, the Rb droplet is created at the top of the cylinder, where the temperature is lower. Thermal simulations indicate a temperature gradient of the order of 10 ° C between the location of the thermistor and the cold spot in the cell. The cold spot temperature defines the vapour pressure and consequently, the atomic density. How to cite this article: Stern, L. et al . Nanoscale light–matter interactions in atomic cladding waveguides. Nat. Commun. 4:1548 doi: 10.1038/ncomms2554 (2013).